Widespread transient Hoogsteen base pairs in canonical duplex DNA with variable energetics Hoogsteen (HG) base pairing involves a 180° rotation of the purine base relative to Watson–Crick (WC) base pairing within DNA duplexes, creating alternative DNA conformations that can play roles in recognition, damage induction and replication. Here, using nuclear magnetic resonance R 1ρ relaxation dispersion, we show that transient HG base pairs occur across more diverse sequence and positional contexts than previously anticipated. We observe sequence-specific variations in HG base pair energetic stabilities that are comparable with variations in WC base pair stability, with HG base pairs being more abundant for energetically less favourable WC base pairs. Our results suggest that the variations in HG stabilities and rates of formation are dominated by variations in WC base pair stability, suggesting a late transition state for the WC-to-HG conformational switch. The occurrence of sequence and position-dependent HG base pairs provide a new potential mechanism for achieving sequence-dependent DNA transactions. We recently showed [1] , [2] , [3] using nuclear magnetic resonance (NMR) R 1ρ relaxation dispersion (RD) [4] , [5] , [6] that A·T and G·C Watson–Crick (WC) base pairs (bps) in CA/TG and TA/TA steps of duplex DNA transiently form Hoogsteen (HG) bps [7] with populations ranging between 0.14 and 0.49% and lifetimes between 0.3 and 2.5 ms at pH ~6 ( Fig. 1a ). HG bps form through 180° rotation of the purine base around the glycosidic bond from an anti to syn conformation ( Fig. 1a ). HG bps modify the structural and chemical presentation of DNA and thereby can play unique roles (reviewed in ref. 8 ) in DNA–protein recognition [9] , [10] , [11] , [12] , damage induction [13] and repair [14] , [15] as well as replication [16] , [17] . For example, by narrowing the minor groove, HG bps have been shown to alter the DNA electrostatic potential ‘seen’ by DNA-binding proteins at the bp edges in the DNA grooves in the context of p53-DNA complexes [12] , [18] , [19] . HG bps can also transiently expose DNA sites that are otherwise inaccessible in WC bps, and thereby provide new mechanisms for damage induction. For example, using computational mapping, Bohnuud et al. [13] recently showed that transient G·C + HG bps could explain the susceptibility and accessibility of cytosines to hydroxymethylation by formaldehyde, thus explaining a long-standing mystery that has persisted for over 25 years. There is also structural and biochemical evidence that some members of the low-fidelity Y-family polymerases replicate DNA using HG pairing as the dominant mechanism, thus providing a mode for bypassing a variety of lesions on the WC face during replication [16] , [17] , [20] . Naked duplexes consisting entirely of HG bps have been reported in A–T-rich sequences that form parallel [21] and anti-parallel stranded [22] , [23] DNA. Computational studies on duplexes also suggest that the HG bp is a reasonable conformation, only slightly less stable than the canonical WC bp [24] , [25] . 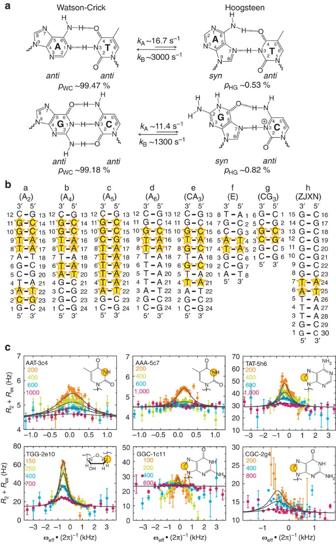Figure 1: Widespread occurrence of transient A·T and G·C+Hoogsteen base pairs in canonical duplex DNA. (a) The equilibrium between Watson–Crick and Hoogsteen base pairs. Shown are the average forward (kA) and reverse (kB) rate constants and populations of Watson–Crick (pA) and Hoogsteen (pB) base pairs obtained in this study. (b) DNA duplexes used in this study. Base pairs targeted for relaxation dispersion measurements are highlighted with a star. (c) Representative off-resonance13C and15NR1ρrelaxation dispersion profiles showing chemical exchange outside TA and CA steps of canonical duplex DNA. Spin lock powers (Hz) are shown in the inset. Data are fit to equation 2. Error bars represent experimental uncertainty (one standard deviation) estimated from monoexponential fitting of duplicateR1ρdata and analysis of signal-to-noise. See Methods for buffer conditions. Figure 1: Widespread occurrence of transient A·T and G·C + Hoogsteen base pairs in canonical duplex DNA. ( a ) The equilibrium between Watson–Crick and Hoogsteen base pairs. Shown are the average forward ( k A ) and reverse ( k B ) rate constants and populations of Watson–Crick ( p A ) and Hoogsteen ( p B ) base pairs obtained in this study. ( b ) DNA duplexes used in this study. Base pairs targeted for relaxation dispersion measurements are highlighted with a star. ( c ) Representative off-resonance 13 C and 15 N R 1ρ relaxation dispersion profiles showing chemical exchange outside TA and CA steps of canonical duplex DNA. Spin lock powers (Hz) are shown in the inset. Data are fit to equation 2. Error bars represent experimental uncertainty (one standard deviation) estimated from monoexponential fitting of duplicate R 1ρ data and analysis of signal-to-noise. See Methods for buffer conditions. Full size image Considering that HG bps are an energetically favourable alternative to WC bps that can provide new mechanisms in a wide variety of DNA biochemical processes, it is of great interest to explore whether the transient HG bps observed by NMR are confined to flexible CA and TA steps, or occur more broadly across distinct sequence and position contexts in duplex DNA. Likewise, it is of interest to examine the sequence specificity of transient HG bp formation as this could provide new mechanisms for achieving sequence-specific DNA transactions that are based on shape [19] . By carrying out 13 C and 15 N R 1ρ NMR RD measurements on 33 bps in eight distinct canonical DNA duplexes, we show that transient HG bps are not limited to CA and TA steps, but rather occur broadly across diverse sequence and positional contexts. We find that both the energetic stability and rates of HG bp formation exhibit a dependence on sequence and position, with HG bps forming faster and being more abundant in energetically less favourable WC bps. Widespread transient HG bps in duplex DNA To more broadly examine the occurrence and sequence specificity of transient HG bps in canonical duplex DNA, we carried out 13 C and 15 N R 1ρ NMR RD measurements targeting sugar C1′ and base C6/8 or N1/3 resonances in 20 A·T and 13 G·C bps in eight DNA duplexes that encompass a variety of sequence motifs, including (A·T) n repeats of varying length ( n =2, 4, 5 and 6), a (CA) 3 repeat, a duplex sequence that forms HG bps on binding to the antibiotic echinomycin, [1] , [26] , [27] a (CG) 3 repeat capable of forming Z-DNA [28] , and a B/Z junction forming sequence [29] , [30] ( Fig. 1b ). The targeted bps ( Fig. 1b , highlighted in stars) encompass 6/10 dinucleotide steps that are positioned 1–6 bps away from the closest terminal end. R 1ρ RD experiments were performed at pH 5.2–7.5 and 5.2–5.4 for A·T and G·C bps, respectively. We use low-pH conditions for transient (and protonated) G·C bps in order to increase the WC-to-HG chemical exchange signature detected by NMR R 1ρ RD [3] . We recently reported a detailed analysis of the pH dependence of chemical exchange corresponding to transient HG bp formation and how measurements at such lower pH conditions can be qualitatively interpolated to assess exchange at higher pH [3] . The R 1ρ NMR RD experiment measures the line broadening contribution to resonances of interest due to chemical exchange with a transient, lowly populated species [4] , [5] . In all cases, we measured significant 13 C and/or 15 N R 1ρ RD ( Supplementary Table 1 ) consistent with chemical exchange ( Fig. 1c and Supplementary Fig. 1 ). A two-state analysis of the R 1ρ data [4] , [5] , [6] (see Methods) yielded populations ( p B =~0.08–2.73%) and lifetimes ( τ B =~0.12–2.57 ms) for the transient state ( Supplementary Fig. 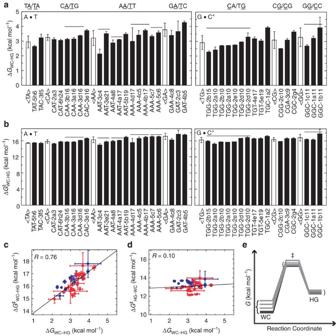Figure 2: Sequence- and position-dependent thermodynamic and kinetic parameters describing the Watson–Crick to Hoogsteen transition. (a) Free-energy difference (ΔGWC−HG) and (b) forward free-energy barrier (ΔG‡WC−HG) for the Watson–Crick to Hoogsteen transition as derived from a two-state analysis of theR1ρdata. Error bars represent experimental uncertainty (one s.d.) estimated from propagation of errors from monoexponential fitting of duplicateR1ρdata and analysis of signal-to-noise. Average and standard deviations for dinucleotide steps are shown using white bars. Horizontal lines denote bps with same triplet sequence and positions relative to nearest terminal end.Xaxis labels denote the triple sequence context (‘XYZ’) with Hoogsteen base pair in the middle; the position relative to the closest terminal end (‘−n’), and name of duplex as denoted inFig. 1b. Correlation between (c) ΔG‡WC−HGand ΔGWC−HGas well as (d) ΔG‡HG−WCand ΔGWC−HG. A·T and G·C+base pairs are shown in red and blue, respectively. The best line of fit and corresponding Pearson coefficient (R) are shown. (e) Free-energy diagram of the Watson–Crick to Hoogsteen transition depicting relative variations in free energy of Watson–Crick, transition and Hoogsteen states. 2 and Supplementary Table 2 ) that are similar to those reported previously for transient HG bps ( p B =~0.14–0.49% and τ B =~0.3–2.5 ms) [1] , [2] . The chemical shifts ( ω B ) of the transient state obtained using this analysis ( Supplementary Fig. 3 and Supplementary Table 2 ) are also consistent with HG bps, including significantly downfield shifted purine C8 (Δ ω ≈2.72 p.p.m. ), purine C1′ (Δ ω ≈3.41 p.p.m. ), cytosine C6 (Δ ω ≈2.40 p.p.m.) and upfield shifted imino N1/3 (Δ ω ≈−1.84 p.p.m.) [1] , [2] . Consistent with HG bps, we did not observe significant chemical exchange at adenine C2 and thymine C6, which do not experience large chemical shift changes upon HG bp formation [1] , [2] ( Supplementary Fig. 1 and Supplementary Table 2 ). These results show that transient HG bps are not confined to CA/TG and TA/TA steps but rather occur broadly across a wide variety of sequence and positional contexts, including G A / T C, A A / T T, T A / T A, G G / C C, C G / C G and TG / CA dinucleotide steps (where the HG bp is underlined). Position- and sequence-dependent energetic variability We observe ~30-fold variations in the transient HG population (0.08–2.73% and 0.13–2.11% for A·T and G·C + bps, respectively) and ~20-fold variations in lifetimes (0.12–2.57 ms and 0.40–2.08 ms for A·T and G·C + bps, respectively) ( Supplementary Fig. 2 and Supplementary Table 2 ). This corresponds to ~2.1 kcal mol −1 and ~2.8 kcal mol −1 variations in the relative thermodynamic stability (ΔΔ G WC–HG with Δ G WC−HG = G HG − G WC ) ( Fig. 2a ) and forward free-energy barriers (ΔΔ G ‡ WC−HG with Δ G ‡ WC−HG = G TS − G WC , where TS is the transition state), respectively ( Fig. 2b ). These variations could reflect real sequence or position dependencies for transient HG bp formation. Alternatively, they could arise due to small differences in buffer conditions used for some of the duplexes (see Methods), particularly pH, which can affect the energetics of transient G·C + HG bp formation [1] , [2] , [3] . However, systematic deviations in Δ G WC−HG and Δ G ‡ WC–HG are not observed across DNA duplexes ( Supplementary Fig. 4a ). Furthermore, no correlations are observed between duplex melting temperatures measured by circular dichroism (CD) ( Supplementary Fig. 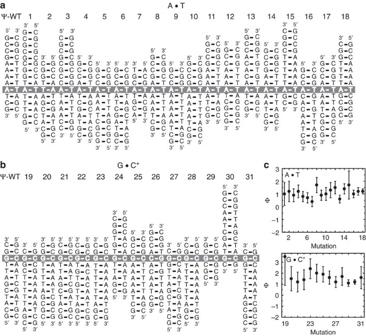Figure 3: Φ-value analysis. Perturbing the Watson–Crick to Hoogsteen equilibrium in (a) A·T and (b) G·C+base pairs by varying the sequence and/or positional context of individual base pairs. All duplexes are re-drawn after aligning each A·T or G·C+base pair with a reference sequence variant (Ψ−WT). (c) Φ-values for A·T and G·C+base pairs. The sequence variant number is shown above each secondary structure. 4b,c and Supplementary Table 3 ) and either Δ G WC−HG or Δ G ‡ WC−HG ( Supplementary Fig. 4a ). Consistent with sequence- and/or position-dependent contributions, the variations in Δ G WC−HG and Δ G ‡ WC−HG are smaller (~1 kcal mol −1 ) when comparing bps across different duplexes that share identical 5′ and 3′ neighbours and positions relative to duplex ends (indicated using horizontal lines in Fig. 2a,b ; Supplementary Fig. 2 and Supplementary Table 2 ). Figure 2: Sequence- and position-dependent thermodynamic and kinetic parameters describing the Watson–Crick to Hoogsteen transition. ( a ) Free-energy difference (Δ G WC−HG ) and ( b ) forward free-energy barrier (Δ G ‡ WC−HG ) for the Watson–Crick to Hoogsteen transition as derived from a two-state analysis of the R 1ρ data. Error bars represent experimental uncertainty (one s.d.) estimated from propagation of errors from monoexponential fitting of duplicate R 1ρ data and analysis of signal-to-noise. Average and standard deviations for dinucleotide steps are shown using white bars. Horizontal lines denote bps with same triplet sequence and positions relative to nearest terminal end. X axis labels denote the triple sequence context (‘XYZ’) with Hoogsteen base pair in the middle; the position relative to the closest terminal end (‘−n’), and name of duplex as denoted in Fig. 1b . Correlation between ( c ) Δ G ‡ WC−HG and Δ G WC−HG as well as ( d ) Δ G ‡ HG−WC and Δ G WC−HG . A·T and G·C + base pairs are shown in red and blue, respectively. The best line of fit and corresponding Pearson coefficient ( R ) are shown. ( e ) Free-energy diagram of the Watson–Crick to Hoogsteen transition depicting relative variations in free energy of Watson–Crick, transition and Hoogsteen states. Full size image We observe significant variations in Δ G WC−HG and Δ G ‡ WC−HG for the same dinucleotide step, which may arise due to differences in position and/or differences in the broader sequence context. Notwithstanding these variations, the average stabilities of HG bps relative to WC bps (ΔG WC−HG ) calculated for individual dinucleotide steps ( Fig. 2a ) follow an order (T A / T A>A A / T T>C A / T G>G A / T C for A·T and T G / C A≥C G / C G≥G G / C C for G·C + ) that is nearly inverted relative to the well-documented WC dinucleotide stabilities (GA/TC≥CA/TG>AA/TT>TA/TA for A·T and CG/CG>GG/CC>TG/CA for G·C), which measure the stability of WC bps relative to the melted state [31] . Thus, transient HG bps seem to be more abundant in less stable WC dinucleotide steps such as CA/TG and TA/TA steps. The energetic preference for HG bps at TA/TA steps observed here is consistent with a large body of data showing that HG bps are favoured in A–T-rich sequences, particularly TA/TA steps (reviewed in ref. 8 ). Origin of variable transient HG bp energetics Strikingly, we observe a clear correlation ( R =0.76) between Δ G WC−HG and Δ G ‡ WC−HG ( Fig. 2c ) and a relatively uniform backward free-energy barrier (Δ G ‡ HG−WC = G TS − G HG ) of ~13 kcal mol −1 ( Fig. 2d ). Thus, changing the sequence context has little effect on the relative energetic stability of the TS and HG bp. This could either be because the stabilities of the TS and HG bp are not significantly affected by changes in sequence, or because their stabilities vary in a correlated manner. In contrast, a change in sequence context does change the relative stability of both the TS and HG bp relative to the WC bp ( Fig. 2e ). One possibility is that sequence-specific variations are dominated by changes in variations in the WC bp without significantly affecting the stabilities of the TS and HG bp ( Fig. 2e ). Indeed, the observed variations in HG bp stability (~2.1 kcal mol −1 ) are comparable in size with variations in WC bp stability (~2 kcal mol −1 ) measured across dinucleotide steps using melting experiments [31] . This would also explain why transient HG bps are specifically more abundant at dinucleotide steps that have weakened WC stabilities ( Fig. 2a,b ). If the observed variations are indeed dominated by variations in WC stability, one might expect a similar correlation between the Δ G cl−op and Δ G ‡ cl−op values describing transitions between WC bps and the bp open state, especially since stability of the open state is not expected to vary significantly with sequence. Indeed, a previous analysis of Δ G cl−op and Δ G ‡ cl−op correlation reported by Coman and Russu [32] based on imino proton exchange measurements [33] reveals a comparably strong correlation ( R =0.8) [34] . Our results suggest that the free energy of the TS varies less relative to the HG bp with sequence/position as compared with the WC bp. If one were to assume that a similar sequence/position-dependent free energy implies a similar structure, even if the sequence/position dependence is very small, then these results would suggest that the TS is structurally more similar to the HG bp—consistent with a ‘late’ TS. Φ-value analysis suggests a ‘late’ transition state To quantify the extent to which the sequence-specific TS energetics are more similar to HG bps versus WC bps, we subjected the measured ΔG WC−HG and Δ G ‡ WC−HG values to Φ-value analysis [34] , [35] (Methods and Fig. 3 ). In this approach, one computes a Φ-value, which quantifies the relative magnitude of the sequence/position-dependent free-energy differences between the TS and WC bps and those between WC bps and HG bps, Figure 3: Φ-value analysis. Perturbing the Watson–Crick to Hoogsteen equilibrium in ( a ) A · T and ( b ) G · C + base pairs by varying the sequence and/or positional context of individual base pairs. All duplexes are re-drawn after aligning each A · T or G · C + base pair with a reference sequence variant (Ψ−WT). ( c ) Φ-values for A · T and G · C + base pairs. The sequence variant number is shown above each secondary structure. Full size image where ΔΔ G TS−WC =( G TS − G WC ) mut −( G TS − G WC ) Ψ−WT and ΔΔ G WC−HG =( G HG − G WC ) mut −( G HG − G WC ) Ψ−WT are the changes in the forward free-energy barrier and free-energy difference between WC and HG bps, respectively, on mutating (mut) the sequence/position of a reference (Ψ−WT) bp. It is instructive to consider two limiting cases to help understand how this analysis can be used to quantify the extent to which the sequence-specific TS energetics are more similar to HG bps versus WC bps and whether a TS is ‘early’ or ‘late’. In the case that the TS and HG share identical sequence-specific energetics as might be expected for a late TS, a given sequence-specific perturbation equally affects G TS and G HG (that is, G HG − G TS =constant for all mutants) and ΔΔ G TS−WC =ΔΔ G WC−HG and Φ=1. On the other hand, if TS and WC share identical sequence-specific energetics as might be expected for an early TS, then G TS – G WC =constant for all mutants and ΔΔ G TS−WC =0 and Φ=0. In practice, the Φ-value can range between 0 and 1, with intermediate Φ-values being more difficult to interpret in the context of a structural mechanism [14] . We arbitrarily assign reference A·T and G·C bps to be those having the smallest Δ G WC −HG values, and which therefore form the most stable HG bps among those studied herein (Ψ−WT, Fig. 3a,b ). Next, we computed Φ for each A·T and G·C + bp. This analysis was preformed separately for A·T and G·C + bps and repeated multiple times assuming a different bp as the designated wild-type reference (data not shown). In the vast majority of the cases, we measure Φ-values near 1, consistent with a ‘late’ TS ( Fig. 3c and Supplementary Table 4 ). It should be noted that similar sequence/position-dependent energetics for the TS and HG bp does not have to imply similarity in structure, and that we cannot rule out the possibility of an early TS that has structural features similar to WC but sequence/position-dependent energetics that are more similar to HG. Our results suggest that HG bps can occur ubiquitously in canonical duplex DNA across different sequence and positional contexts. This can help explain how polymerases such as the human DNA polymerase iota can use HG pairing as a general mechanism to replicate DNA and thereby bypass lesions that diminish the ability to form WC bps [8] , [16] . Our findings also raise the possibility that HG bps may be widespread in genomic DNA, especially given that the energetic differences between WC and HG bps are small compared with forces in living cells, including those arising due to supercoiling, torsional stress, and protein binding. It is worth noting that difficulties in distinguishing between WC and HG bps based on X-ray crystallography data have been reported [8] , [36] . Our finding that transient HG bps can occur ubiquitously in duplex DNA calls for the re-examination of current X-ray structures of DNA to more critically assess for the occurrence of HG bps. Our studies suggest that the occurrence of HG bps depends in a complex manner on both sequence context and position. This is consistent with the hypothesis by Honig and Rohs [37] that the observation of HG base pairing makes it is unlikely that protein–DNA binding is driven by a simple linear code. Nevertheless, our results together with prior studies [8] suggest that HG bps are likely to exist in greater abundance within unstable and structurally stressed environments, such as kinks and turns, which can destabilize WC bps, including stacking interactions. Indeed, while only a few X-ray structures have documented the existence of HG bps in DNA, in many cases HG bps occur near structurally stressed environments. For example, HG bps are observed near kinks or nicks in X-ray structures of DNA bound to TATA box-binding protein [11] and integration host factor [9] , and near a hairpin loop in structures of DNA bound to TnpA transposase [38] . HG bps have also been observed for DNA in complex with antibiotics that contribute unique stacking interactions [27] , [39] . Previous studies [3] have shown that changes in counterion concentration have a measurable effect on the population and lifetime of HG bps. Future studies should therefore also examine how the sequence- and position-dependent HG energetics vary with increasing counterion concentration (Na + and Mg 2+ ). Studies so far suggest that Na + and Mg 2+ stabilize A·T HG but destabilize G·C + HG bps in the case of CA/TG steps [3] . Although further studies are needed to more quantitatively understand the sequence and position dependence of transient HG bp formation, these energetic preferences may provide a new mechanism for shape-based DNA recognition [12] , [19] via indirect read-out mechanisms [40] . Our study has focused on the occurrence of single transient HG bps surrounded by WC bps. Additional studies are needed to examine sequence-specific propensities for forming longer stretches of HG bps, and HG tracts interspersed by WC bps. Such mixtures of WC and HG bps can endow genomic DNA with a new level of structural complexity similar to Z-DNA. Our results suggest that the sequence- and position-specific variations in HG bp stabilities and lifetimes are dominated by variations in the WC bp stability and to a lesser extent by variations in the stabilities of the TS and HG bp. Interestingly, a similar trend has been reported for base opening [32] . Future studies should further explore the WC-to-HG transition pathways and examine whether they share a similar TS with base opening and whether there can be pathways toward HG that proceed via the base-opened state. Conjugate peak refinement simulations suggest a pathway in which the purine base rotates toward the major groove inside the double helix [1] ; however, further experimental characterization is required. The observation that the sequence and/or position variations in the TS free energies are more similar to the HG bp versus the WC bp suggests the TS is structurally more similar to HG versus WC, consistent with a ‘late’ TS for the WC-to-HG transition. However, we cannot rule out an early TS that is structurally more similar to WC but has sequence/position-dependent energetics that are more similar to the HG bp. Although the structure of the TS remains unclear, an equally important question is why the energetic stabilities of HG bps appear to be only weakly dependent on sequence. Further studies are required to understand the structure and specific interactions that may help stabilize the TS and HG bp. NMR samples and resonance assignments Unlabelled DNA samples were purchased as single-stranded oligos from Integrated DNA Technologies (IDT) with standard desalting purification. The DNA oligos were resuspended to ~200 μM in 15 mM phosphate buffer with corresponding pH (see below), 25 mM NaCl, 0.1 mM EDTA. Duplexes were annealed by mixing an equimolar ratio of the complementary DNA strands, heating at 95 °C for 2 min followed by gradual cooling at room temperature for ~30 min. Unlabelled DNA duplexes were washed 3 × in resuspension buffer by microcentrifugation using an Amicon Ultra-4 centrifugal filter with a 3-kDa cutoff, concentrated to ~2–3 mM and ~250 μl, then supplied with 10% D 2 O. Natural abundance CG 3 was resuspended in~4 ml of milliQ H 2 O and dialyzed against 2 l of milliQ H 2 O with two exchanges for a total of 6 l of milliQ H 2 O, using a dialysis tube from G-Biosciences with a 1-kDa cutoff. Dialyzed CG 3 was lyophilized and resuspended in NMR buffer to ~4 mM and supplied with 10% D 2 O. Hemi- 13 C/ 15 N-labelled A 5 duplex was prepared by annealing a uniformly 13 C/ 15 N-labelled thymine-rich strand to a natural abundance adenosine-rich strand. Fully 13 C/ 15 N-labelled DNA duplexes were prepared by annealing two labelled strands together. All labelled single strands were synthesized in vitro by the method of Zimmer and Crothers [41] using a DNA hairpin template with a 5′ overhang corresponding to the complement of the target labelled strand and a 3′ ribose (IDT). In this study, we used the same hairpin sequence as Zimmer and Crothers [41] , Klenow fragment DNA polymerase (NEB) NEB2 buffer (NEB) and uniformly 13 C/ 15 N-labelled dNTPs (Isotec, Sigma-Aldrich and Silantes). Base- and heat-catalyzed cleavage separated the hairpin template from the 13 C/ 15 N-labelled synthesized product. The single-stranded DNA product was purified by 20% denaturing polyacrylamide gel electrophoresis, isolated by passive elution from crushed gel pieces and desalted on a C18 reverse-phase column (Sep-Pak, Waters). The oligo was lyophilized and suspended in NMR buffer. The semi-labelled DNA samples were prepared by titrating the unlabelled strand directly into an NMR tube containing the 13 C/ 15 N-labelled strand and monitoring the disappearance of single-stranded DNA peaks using heteronuclear single quantum coherence (HSQC) experiments. The fully labelled samples were annealed in a similar fashion. 2D 1 H– 1 H nuclear overhauser spectroscopy (NOESY) experiments at 26 °C (A 2 , A 4 , A 5 , A 6 , CA 3 , E) or 25 °C (CG 3 and Z junction (ZJXN)) and pH 5.2 (A 5 ), 5.4 (A 2 , A 4 , A 6 , CA 3 , CG 3 ), 6.8 (E) or 7.5 (ZJXN) were used to assign resonances as described previously [1] . See NMR R 1ρ relaxation dispersion for R 1ρ RD pH values. NMR R 1ρ RD All NMR experiments were performed on a Bruker Avance 600 MHz NMR spectrometer equipped with a 5-mm triple-resonance cryogenic probe. R 1ρ RD experiments were performed at pH 5.2–7.5 and 5.2–5.4 for A·T and G·C + bps, respectively. Buffer conditions for R 1ρ RD measurements are 15 mM sodium phosphate, 25 mM NaCl, 0.1 mM EDTA, 10% D 2 O pH=5.2 (A 5 , A 4 : C15 C6, A16 C1′, G10 C1′), pH=5.4 (A 2 , A 4 , A 6 , CA 3 , CG 3 ), pH=6.8 (E) and pH=7.5 (ZJXN) at 26 °C (A 2 , A 4 , A 5 , A 6 , CA 3 , E) or 25 °C (A 2 A3 C1′, CG 3 , ZJXN). CG 3 and E are unlabelled DNA samples, the T-rich strand of A 5 is 13 C/ 15 N labelled while A 6 , A 4 , A 2 , CA 3 and ZJXN are fully 13 C/ 15 N-labelled. We use low-pH conditions for transient (and protonated) G·C + bps in order to increase the WC-to-HG chemical exchange signature detected by R 1ρ RD [3] . We recently reported a detailed analysis of the pH dependence of chemical exchange corresponding to transient HG bp formation and how measurements at such lower pH conditions can be qualitatively interpolated to assess exchange at higher pH [3] . Carbon and nitrogen R 1ρ RD profiles for guanine/adenine C8, guanine/adenine C1′, cytosine C6, guanine N1 and thymine N3 were measured using a one-dimensional acquisition scheme which uses selective Hartmann–Hahn polarization transfer [42] to selectively excite one C–H or N–H spin system at a time [6] . The spin lock power and offset frequencies are summarized in Supplementary Table 4 . The following delays were used: A 2 : A3 C1′, G10 C1′, A17 C1′; A 4 : A5 C1′, G10 C1′, A16 C1′, A19 C1′; CA 3 : G10 C1′; A 5 : A3 C1′, C5 C1′ (0, 4, 8, 12, 18, 26, 34, 42, 12, 42); A 5 G11 C8 (0, 12, 32, 26, 32); A 4 A17 C8, A 6 A17 C8 (0, 4, 12, 32, 26, 32); A 2 : C2 C6, T9 C6, G11 C8, A16 C8, A17 C2; CA 3 : A16 C8, C17 C6, C19 C6, A21 C1′; A 4 : C15 C6, G11 C8; A 5 : C9 C6, G10 C8; A 6 : G10 C8, A16 C8 (0, 4, 8, 12, 16, 20, 26, 32, 12, 32); A 2 : T8 N3, G10 N1, G23 N1; A 5 : T4 N3, T5 N3, T6 N3, T7 N3, T8 N3; A 6 G10 N1 (0, 8, 16, 24, 36, 48, 60, 80, 100, 16, 70, 100); CG 3 G4 C8 (0, 60, 60); ZJXN: A6 C8, A24 C8 (0, 4, 8, 12, 16, 20, 24, 30, 12, 30); E A5 C8: (0, 48, 48). Data points meeting C-C Hartmann–Hahn matching conditions were omitted as described previously [6] . Data were processed using NMRPipe [43] and R 1ρ values were determined from monoexponential decay fits of the resonance intensities using a script [44] in Mathematica 9 (Wolfram Research). On- and off-resonance R 1ρ data were fit to the Laguerre equation [45] (equation 2) using Origin 8.6 (OriginLab), Where , and . Δ ω AB =Ω B −Ω A , where Ω A and Ω B are the chemical shifts of the ground (A) and transient (B) states, respectively, in Hz. R 1 and R 2 are the intrinsic longitudinal and transverse relaxation rate constants, respectively, and are assumed to be identical for the ground (A) and transient (B) states. θ =arctan( ω 1 /Ω) where ω 1 is the spin lock power strength. Ω=Ω obs − ω rf where Ω is the offset of the spin lock carrier frequency ( ω rf ) from the observed resonance frequency (Ω obs ). Ω obs = p A Ω A + p B Ω B where p A and p B are the ground and transient state populations, respectively, and p A + p B =1. k ex is the chemical exchange rate constant for a two-state exchange process where k ex = k A + k B , k A = k ex p B and k B = k ex p A . k A and k B are the forward and reverse rate constants, respectively. Plots of R 1ρ data are presented as R 2eff ( R 2eff = R 2 + R ex ) in Fig. 1c and Supplementary Fig. 1 where, In cases where large errors were accompanied by small R ex , model selection comparing presence and absence of exchange was carried out using the F- and Akaike’s Information Criterion (AIC) [46] tests to discriminate between exchange and no detectable exchange (data not shown). The F-test compares two nested models fit to the same data under the null hypothesis that the residual sum of squares of the less complex, restricted model is not significantly larger than that of the more complex, full model. The AIC test assesses the likelihood of a model given the data and seeks to minimize loss of information embedded within the data. For A 2 G23 N1, no exchange is the selected model under the conditions used. Because of lower sensitivity to exchange, we did not interpret absence of 15 N dispersion as evidence for absence of transient HG bps. The free-energy difference between the WC GS and HG transient state (Δ G WC−HG ) was computed using, where k 1 and k 2 are the forward and reverse rate constants, respectively, h is Planck’s constant, k B is Boltzmann’s constant, R is the gas constant and T is temperature. The forward barrier of the transition (Δ G ‡ WC−HG ) was computed using, where κ is the transmission coefficient which is assumed to be unity. CD melting DNA duplexes (IDT) were prepared using ultracentrifugation as described in NMR Samples and Resonance Assignments in 15 mM phosphate buffer, 0.1 mM EDTA, 25 mM NaCl pH 5.4 and supplied with 10% D 2 O. Duplexes were prepared by diluting complementary single-stranded stocks to 50 μM in the same tube with a final volume of 200 μl. Samples were denatured at 95 °C for 5 min followed by annealing of at least 10 min on the bench top. Samples were transferred to a 1-mm cuvette (Starna Cells), mineral oil was added to the top of the solution and the cuvette was capped. Melting experiments were performed on a Jasco Spectropolarimeter equipped with a recirculating water bath and Peltier temperature control unit. Temperature ramps were performed from 5 to 80 °C with a bandwidth of 5 nm (1 nm for ZJXN), ramp rate of 1 °C min −1 , equilibration time of 20 s and sensitivity of 100 millidegrees. Wavelength scans used the same sensitivity and bandwidth as melting runs. Spectral measurements were performed between 220 to 330 nm with a scan rate of 100 nm min −1 . Temperature ramp profiles were fit to the Boltzmann model [47] , which has previously been used to determine nucleic acid melting temperatures [48] , where θ is the elipticity at 254 nm normalized to the signal change magnitude, LL and UL are the lower and upper limits of the transition, respectively, a is the Hill slope, T m is the melting temperature defined as the point of inflection of the melting curve and T is the independent variable temperature. Phi (Φ)-value analysis Φ-value analysis [34] was carried out by computing Φ using equation 1 (Φ=ΔΔ G TS−WC /ΔΔ G WC−HG ) where ΔΔ G TS−WC =Δ G ‡ WC−HG,mut −Δ G ‡ WC−HG,Ψ−WT and ΔΔ G WC−HG =Δ G WC–HG,mut −Δ G WC−HG,Ψ−WT are the change in the forward free-energy barrier (Δ G ‡ WC−HG ) and free-energy difference between WC and HG bps (Δ G WC−HG ), respectively, on introduction of one or multiple mutations (mut) as compared with ‘wild-type’ (Ψ−WT). We defined Ψ-WT to be A 5 T4 N3 and A 2 G10 N1 for A·T and G·C + bps, respectively, given that they have the lowest ΔG WC−HG values. To control for systematic errors in Φ arising due to use of a 15 N Ψ−WT reference resonance, we also performed Φ-value analysis assigning a 13 C resonance as Ψ−WT for A·T and G·C + bps, respectively. In all cases we observe Φ-values concentrated around ~1 consistent with a ‘late’ TS. Note that Φ≈ 0 when ΔΔ G TS−WC ≈0 relative to ΔΔ G WC−HG implying an early WC-like TS, whereas Φ≈1 when ΔΔ G TS−WC ≈ΔΔ G WC−HG and implies a late HG-like TS. Errors for calculated Φ-values for A 6 A17 C8, A 2 A3 C1′, A 4 C15 C6 and A 5 G10 C8 were larger than the corresponding values and thus could not be determined accurately. How to cite this article: Alvey, H. S. et al. Widespread transient Hoogsteen base pairs in canonical duplex DNA with variable energetics. Nat. Commun. 5:4786 doi: 10.1038/ncomms5786 (2014).